SLO-2 potassium channel is an important regulator of neurotransmitter release inCaenorhabditis elegans Slo2 channels are prominent K + channels in mammalian neurons but their physiological functions are not well understood. Here we investigate physiological functions and regulation of the Caenorhabditis elegans homologue SLO-2 in motor neurons through electrophysiological analyses of wild-type and mutant worms. We find that SLO-2 is the primary K + channel conducting delayed outward current in cholinergic motor neurons, and one of two K + channels with this function in GABAergic motor neurons. Loss-of-function mutation of slo-2 increases the duration and charge transfer rate of spontaneous postsynaptic current bursts at the neuromuscular junction, which are physiological signals used by motor neurons to control muscle cells, without altering postsynaptic receptor sensitivity. SLO-2 activity in motor neurons depends on Ca 2+ entry through EGL-19, an L-type voltage-gated Ca 2+ channel (Ca V 1), but not on other proteins implicated in either Ca 2+ entry or intracellular Ca 2+ release. Thus, SLO-2 is functionally coupled with Ca V 1 and regulates neurotransmitter release. A major function of K + channels in neurons is to regulate the release of neurotransmitters. A variety of K + channels have been found to have this physiological function, including the Ca 2+ - and voltage-gated high-conductance K + channel Slo1 (BK channel) [1] . Recent studies show that two other large-conductance K + channels of the Slo gene family, Slo2.2 ( Slack ) and Slo2.1/ Slick , are also broadly expressed in the nervous system [2] , [3] ( www.brain-map.org ). Slo2.2 plays major roles in conducting delayed outward current in diverse mammalian central neurons examined [4] , [5] , [6] . Suppression of Slo2.2 expression may enhance neuron excitability and pain sensitivity [7] , [8] , [9] . A strong link has been established between mutations of KCNT1 (gene encoding Slo2.2) and epileptic disorders [10] , [11] , [12] , [13] , [14] . These observations suggest that Slo2 channels in neurons may play important physiological roles. However, studies on Slo2 channels with either knockout preparations or specific blockers are lacking, which makes it difficult to precisely define their physiological roles. Slo2 channels are activated by membrane depolarization and cytosolic Cl − and Na + (refs 15 , 16 ). They are considered to be the molecular entity of Na + -activated K + (K Na ) channels observed in a variety of cells [17] , [18] . One conundrum about K Na channels is that a concentration of Na + much higher than what could possibly occur in the bulk cytoplasm under physiological conditions is required for significant channel activation [17] , [18] , although these channels appear to be active under physiological conditions [5] , [19] , [20] , [21] . Recent studies of Slo2.2 suggest that Na + entry, through either a persistent tetrodotoxin-sensitive channel(s) of unknown molecular identity [4] , [5] , [6] or AMPA receptors [22] , may produce Na + microdomains necessary for K Na channel activation. Caenorhabditis elegans has a single Slo2 orthologue known as SLO-2, which is also gated by voltage and intracellular Cl − but differs from mammalian Slo2 in that intracellular Ca 2+ instead of Na + activates the channel [23] , [24] . The [Ca 2+ ] required for C. elegans SLO-2 activation [23] is also much higher than what could possibly occur in the bulk cytoplasm under physiological condition. It is unknown whether Ca 2+ entry plays an analogous role in SLO-2 activation as does Na + entry for Slo2 activation. In C. elegans body-wall muscle, SLO-2 conducts ~70% of the total delayed outward current, and slo-2 loss-of-function ( lf ) mutation results in a more depolarized resting membrane potential, a wider action potential waveform and a smaller amplitude of afterhyperpolarization, suggesting that SLO-2 plays important roles in controlling muscle function [25] . Although SLO-2 is also expressed in the nervous system [23] , [26] , its physiological roles in neurons are unknown. C. elegans neuromuscular junction (NMJ) is often used as a model synapse for analysing the roles of proteins in synaptic transmission. However, electrophysiological analyses of this synapse have been limited to recording postsynaptic current (PSC) from body-wall muscle cells. To our knowledge, there has been no report on whole-cell voltage- and current-clamp recordings from C. elegans motor neurons. In the present study, we successfully performed electrophysiological recordings of motor neurons, and combined the electrophysiological data with PSCs recorded from body-wall muscle cells to assess physiological roles of SLO-2 in motor neurons. Our results suggest that SLO-2 is a major contributor to delayed outward current in motor neurons with its activity dependent on Ca 2+ entry through a L-type voltage-gated Ca 2+ channel (VGCC), and that SLO-2 controls the strength of synaptic transmission by regulating the duration and charge transfer rate of PSC bursts, which are used by motor neurons to control body-wall muscle [27] . The prominent roles of Slo2/SLO-2 in conducting delayed outward current in both mammalian and nematode neurons suggest that these channels likely have important and conserved physiological functions. SLO-2 is important to outward current in motor neurons Motor neurons controlling C. elegans body-wall muscle include the following three major classes: A, B and D. The A and B classes mediate backward and forward movements, respectively, and contract muscle by releasing acetylcholine (ACh), whereas the D class relaxes muscle by releasing GABA (γ-aminobutyric acid) [28] , [29] . To investigate physiological roles of SLO-2 in motor neurons, we chose VA5, VB6 and VD5 (the letter ‘V’ stands for ventral) as representatives of the three classes of motor neurons because these ventral muscle-innervating neurons could be easily identified based on their anatomical locations ( Fig. 1a ). We first examined the effect of slo-2 mutation on delayed outward current in response to voltage steps (−60 to +70 mV at 10-mV intervals). The amplitude of delayed outward current was greatly decreased in slo-2(nf101) , a putative null resulting from a deletion [30] , compared with wild type (WT) in all the motor neurons ( Fig. 1b ). The decrease was more severe in VA5 and VB6 than VD5. Compared with WT, delayed outward current at +70 mV decreased by 80% in VA5 (168.9±16.6 versus 33.6±2.4 pA/pF), 67% in VB6 (176.1±13.4 versus 58.1±3.1 pA/pF) and 33% in VD5 (197.1±12.5 versus 131.9±5.6 pA/pF) ( Fig. 1b ). The deficiency of delayed outward current in the mutant was rescued by expressing a SLO-2::GFP fusion protein, in which GFP coding sequence was fused in-frame to the 3′-end of slo-2b (F08B12.3b) cDNA ( www.wormbase.org ) [23] , under the control of the pan-neuronal rab-3 promoter (P rab-3 ; refs 31 , 32 ; Fig. 1b ), suggesting that the deficiency resulted from slo-2 mutation in neurons, and that the SLO-2::GFP fusion protein was functional. 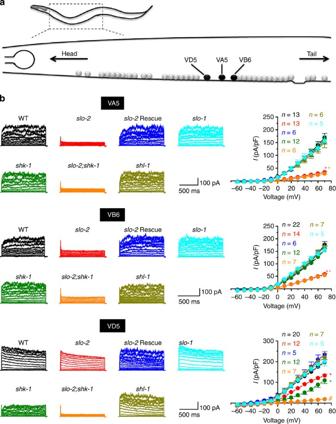Figure 1: SLO-2 is an important contributor to delayed outward current in cholinergic and GABAergic motor neurons. (a) Diagram showing the locations of the recorded motor neurons VD5, VA5 and VB6 (based on published anatomical data63). (b) Sample whole-cell current traces in response to voltage steps (−60 to +70 mV at 10 mV intervals) from a holding voltage of −60 mV (left) and current–voltage relationships (right) from VA5, VB6 and VD5 of WT,slo-2(nf101),slo-2rescue, shk-1(ok1581), slo-2(nf101);shk-1(ok1581),shl-1(ok1168)andslo-1(md1745). In VA5 and VB6, delayed outward current was greatly decreased inslo-2(nf101)compared with WT but not further decreased in theslo-2;shk-1double mutant. In VD5, delayed outward current was greatly decreased in bothslo-2(nf101)andshk-1(ok1581), and was essentially absent in theslo-2;shk-1double mutant. Data are shown as mean±s.e. The asterisk (*) indicates a significant difference compared with WT, whereas the pound sign (#) indicates a significant difference compared with the single mutants ofslo-2andshk-1(P<0.01, two-way mixed model analyses of variance with Tukey’spost hoctests). The recordings were performed with extracellular solution I and pipette solution I. Figure 1: SLO-2 is an important contributor to delayed outward current in cholinergic and GABAergic motor neurons. ( a ) Diagram showing the locations of the recorded motor neurons VD5, VA5 and VB6 (based on published anatomical data [63] ). ( b ) Sample whole-cell current traces in response to voltage steps (−60 to +70 mV at 10 mV intervals) from a holding voltage of −60 mV (left) and current–voltage relationships (right) from VA5, VB6 and VD5 of WT, slo-2(nf101) , slo-2 rescue , shk-1(ok1581), slo-2(nf101);shk-1(ok1581) , shl-1(ok1168) and slo-1(md1745) . In VA5 and VB6, delayed outward current was greatly decreased in slo-2(nf101) compared with WT but not further decreased in the slo-2;shk-1 double mutant. In VD5, delayed outward current was greatly decreased in both slo-2(nf101) and shk-1(ok1581) , and was essentially absent in the slo-2;shk-1 double mutant. Data are shown as mean±s.e. The asterisk (*) indicates a significant difference compared with WT, whereas the pound sign ( # ) indicates a significant difference compared with the single mutants of slo-2 and shk-1 ( P <0.01, two-way mixed model analyses of variance with Tukey’s post hoc tests). The recordings were performed with extracellular solution I and pipette solution I. Full size image The persistence of some delayed outward current in slo-2(nf101) suggests that there is at least one more K + channel functioning in motor neurons. It is difficult to do a comprehensive survey for the many voltage-gated K + channels existing in C. elegans [33] . Previous studies show that three voltage-gated K + channels are important to outward current in C. elegans body-wall muscle cells, including SLO-2, SHK-1 ( Shaker or K V 1) and SHL-1 ( Shal or K V 4), with SLO-2 and SHK-1 conducting delayed outward current and SHL-1 conducting a fast and transient outward current [25] , [34] , [35] . This knowledge was used as a guide in identifying the remaining K + channel(s) contributing to outward current in motor neurons. SLO-1, the C. elegans Slo1/BK channel, was also included in our analyses because it is expressed in C. elegans motor neurons and plays an important role in regulating neurotransmitter release [36] . The mutants analysed included shk-1(ok1581) , shl-1(ok1168) and slo-1(md1745) , which are all putative nulls [25] , [35] , [36] . Delayed outward current was normal in VA5 and VB6 of all the mutants ( Fig. 1b ) but greatly decreased in VD5 of shk-1(ok1581) ( Fig. 1b ). In fact, delayed outward current of VD5 was decreased to a larger degree in shk-1(ok1581) (45%) than slo-2(nf101) (33%) at +70 mV (WT 197.1±12.5 pA/pF; shk-1 108.9±15.6 pA/pF; slo-2 131.9±5.6 pA/pF) and was essentially absent in the double mutant ( Fig. 1b ). Collectively, the aforementioned observations suggest that delayed outward current of VA5 and VB6 results primarily from SLO-2 with a small contribution from an unidentified channel(s), whereas that of VD5 results almost completely from SHK-1 and SLO-2. SLO-2 regulates membrane potential of motor neurons In WT worms, the resting membrane potential was −71.7±2.4 mV in VA5, −53.2±2.5 mV in VB6 and −45.8±1.9 mV in VD5. It became significantly less hyperpolarized in slo-2(nf101) but was restored to WT level in the slo-2(nf101) strain expressing P rab-3 ::SLO-2::GFP ( Table 1 ). In contrast, mutants of the other K + channels did not show a change of the resting membrane potential compared with WT ( Table 1 ). These observations suggest that SLO-2 plays an important role in setting the resting membrane potential of both cholinergic and GABAergic motor neurons. Table 1 Comparison of the resting membrane potential of motor neurons between wild type and K + channel mutants. Full size table To assess the role of SLO-2 in regulating motor neuron activity, we analysed spontaneous membrane voltage changes of VA5. In both WT and slo-2(nf101) , the membrane voltage alternated between the resting membrane potential and an upstate, with apparent spontaneous postsynaptic potentials decorating both periods ( Fig. 2a ). The upstate often reached a similar level in each recording and never overshot ( Fig. 2a ). Compared with WT, the upstate of slo-2(nf101) was 61% smaller in amplitude (33.4±1.4 versus 13.1±0.9 mV) and 45% longer in duration (14.9±1.5 versus 21.6±2.6 s) without a change in frequency ( Fig. 2b ). Since upstate potential (the mean membrane potential during the upstate) was similar between WT and slo-2(nf101) ( Fig. 2b ), the smaller upstate amplitude of the mutant resulted from the elevated resting membrane potential. 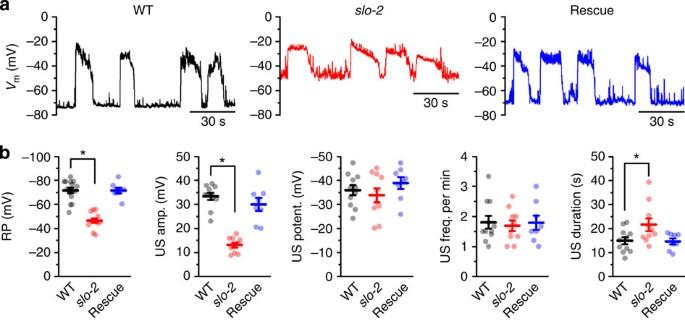Figure 2: Loss-of-function mutation ofslo-2reduced the amplitude of a spontaneous upstate in motor neurons. (a) Samples traces of spontaneous membrane voltage changes of VA5 from wild type (WT),slo-2(nf101)andslo-2(nf101)rescued by expressing WT SLO-2b under the control of Prab-3. (b) Comparison of the resting membrane potential (RP) and upstate (US) frequency (freq.), duration, amplitude (amp.) and potential (potent.). Both the averaged value of each experiment (filled circle) and the mean±s.e. of the group (line and bar) are shown. The asterisk (*) indicates a statistically significant difference compared with WT (P<0.05, one-way analyses of variance with Tukey’spost hoctests). The sample size (n) was 15 for WT, 12 forslo-2and 8 for Rescue. Samples without obvious USs (four WT and twoslo-2mutant) were not included in the US quantifications. The recordings were performed with extracellular solution I and pipette solution I. Figure 2: Loss-of-function mutation of slo-2 reduced the amplitude of a spontaneous upstate in motor neurons. ( a ) Samples traces of spontaneous membrane voltage changes of VA5 from wild type (WT), slo-2(nf101) and slo-2(nf101) rescued by expressing WT SLO-2b under the control of P rab-3 . ( b ) Comparison of the resting membrane potential (RP) and upstate (US) frequency (freq. ), duration, amplitude (amp.) and potential (potent.). Both the averaged value of each experiment (filled circle) and the mean±s.e. of the group (line and bar) are shown. The asterisk (*) indicates a statistically significant difference compared with WT ( P <0.05, one-way analyses of variance with Tukey’s post hoc tests). The sample size ( n ) was 15 for WT, 12 for slo-2 and 8 for Rescue. Samples without obvious USs (four WT and two slo-2 mutant) were not included in the US quantifications. The recordings were performed with extracellular solution I and pipette solution I. Full size image SLO-2 regulates neurotransmitter release To determine whether SLO-2 in motor neurons regulates synaptic transmission, we analysed spontaneous and evoked PSCs at the C. elegans NMJ. We first focused on spontaneous PSC bursts, defined as an apparent increase in PSC frequency with a persistent current lasting >3 s, because they are the physiological signals used by motor neurons to control muscle contractility [27] . The persistent current, appearing as an apparent downward shift of the baseline, was used to demarcate PSC bursts, as described previously [27] . Cholinergic PSC bursts were isolated by using pipette and extracellular solutions with the Cl − equilibrium potential equal to the holding potential (−60 mV). Compared with WT, slo-2(nf101) showed significantly longer duration and higher charge transfer rate in PSC bursts, which were restored to WT level when SLO-2::GFP was expressed in neurons ( Fig. 3a,b ). The main cause for the higher charge transfer rate of PSC bursts in slo-2(nf101) was a larger mean persistent current because amplitude of the persistent current increased by 87% (WT 4.6±0.5 pA; slo-2 8.6±0.8 pA) ( Fig. 3b ) but frequency and amplitude of intra-burst PSC events were unaltered compared with WT ( Fig. 3c ). 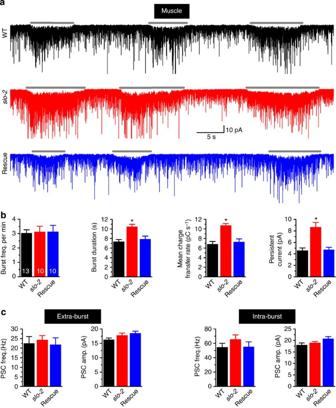Figure 3: SLO-2 deficiency augmented PSC bursts recorded from body-wall muscle. (a) Representative traces of spontaneous PSC. The horizontal grey line marks PSC bursts. (b) Comparison of PSC burst properties. (c) Comparison of extra- and intra-burst PSC events. The sample sizes (n) were 17 for wild type (WT), 15 forslo-2(nf101) and 10 forslo-2(nf101) expressing Prab-3::SLO-2::GFP (Rescue). Data are shown as mean±s.e. The asterisk (*) indicates a statistically significant difference compared with WT (P<0.05, one-way analyses of variance with Tukey’spost hoctests). The recordings were performed with extracellular solution I and pipette solution II. Amp., amplitude; freq., frequency. Figure 3: SLO-2 deficiency augmented PSC bursts recorded from body-wall muscle. ( a ) Representative traces of spontaneous PSC. The horizontal grey line marks PSC bursts. ( b ) Comparison of PSC burst properties. ( c ) Comparison of extra- and intra-burst PSC events. The sample sizes ( n ) were 17 for wild type (WT), 15 for slo-2 ( nf101 ) and 10 for slo-2 ( nf101 ) expressing P rab-3 ::SLO-2::GFP (Rescue). Data are shown as mean±s.e. The asterisk (*) indicates a statistically significant difference compared with WT ( P <0.05, one-way analyses of variance with Tukey’s post hoc tests). The recordings were performed with extracellular solution I and pipette solution II. Amp., amplitude; freq., frequency. Full size image The larger persistent current of cholinergic PSC bursts observed in slo-2(nf101) could have resulted from either increased neurotransmitter release or increased postsynaptic receptor sensitivity to ACh. To examine the second possibility, we compared the amplitude of inward current caused by pressure-ejecting exogenous ACh (100 μM) to body-wall muscle cells between WT and slo-2(nf101) . A similar experiment with exogenous GABA (100 μM) was also performed although GABA did not contribute to the PSC bursts under the experimental conditions [27] . We found that amplitudes of ACh- and GABA-induced inward current were similar between WT and slo-2(nf101) ( Fig. 4a ). Thus, the larger persistent current of PSC bursts in slo-2(nf101) did not result from an increased postsynaptic receptor function or expression. 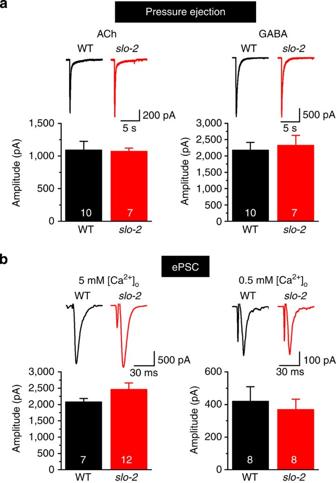Figure 4: Postsynaptic receptor sensitivities and evoked postsynaptic currents (ePSCs) were normal inslo-2(nf101). (a) Comparison of muscle cell response to pressure-ejected acetylcholine (ACh; 100 μM) or GABA (100 μM) between wild type (WT) andslo-2(nf101). (b) Comparison of ePSC between WT andslo-2(nf101)in the presence of two different extracellular Ca2+concentrations (5 and 0.5 mM). Data are shown as mean±s.e. No significant difference was detected (unpairedt-test). The holding voltage was −60 mV in all the experiments. The numbers inside the columns indicate the sample sizes (n). All the recordings were performed with pipette solution I. The recordings of ePSC at 0.5 mM [Ca2+]owere performed with extracellular solution II, whereas the remaining recordings were recorded with extracellular solution I. Figure 4: Postsynaptic receptor sensitivities and evoked postsynaptic currents (ePSCs) were normal in slo-2(nf101) . ( a ) Comparison of muscle cell response to pressure-ejected acetylcholine (ACh; 100 μM) or GABA (100 μM) between wild type (WT) and slo-2(nf101) . ( b ) Comparison of ePSC between WT and slo-2(nf101) in the presence of two different extracellular Ca 2+ concentrations (5 and 0.5 mM). Data are shown as mean±s.e. No significant difference was detected (unpaired t -test). The holding voltage was −60 mV in all the experiments. The numbers inside the columns indicate the sample sizes ( n ). All the recordings were performed with pipette solution I. The recordings of ePSC at 0.5 mM [Ca 2+ ] o were performed with extracellular solution II, whereas the remaining recordings were recorded with extracellular solution I. Full size image We also compared evoked PSCs (ePSCs) caused by electric stimulation of motor neurons between WT and slo-2(nf101) . Evoked PSCs were analysed in the presence of two different [Ca 2+ ] o (5 and 0.5 mM) because an effect of slo-2 mutation on the evoked responses could potentially vary depending on [Ca 2+ ] o , as is the case with slo-1 mutation [37] . We found that evoked PSCs were similar in amplitude between WT and slo-2(lf) in the presence of either 5 or 0.5 mM [Ca 2+ ] o ( Fig. 4b ), suggesting that SLO-2 does not regulate neurotransmitter release caused by strong non-physiological stimuli. SLO-2 in motor neurons requires Cl − and Ca 2+ for activation Analyses with inside-out patches from Xenopus oocytes show that SLO-2 has a mean single-channel conductance of 110 pS in symmetrical K + , and is activated synergistically by Ca 2+ and Cl − on the intracellular side [23] . However, single-channel conductance of SLO-2 in neurons has not been reported, the concentration of free Ca 2+ required for significant SLO-2 activity [23] is much higher than what could possibly be reached in the bulk cytoplasm under physiological conditions, and the reported Cl − sensitivity of SLO-2 was rebutted by a recent study [38] . We therefore performed experiments to assess the single-channel conductance of SLO-2 in motor neurons and to determine whether SLO-2 in motor neurons is sensitive to Ca 2+ and Cl − . First, we recorded SLO-2 single-channel activities in inside-out patches held at a series of voltages in the presence of symmetrical K + solutions to determine SLO-2 single-channel conductance. In WT, each patch typically showed activities of a few channels, which were apparently of the same type ( Fig. 5a ). In contrast, similar single-channel opening events were never observed in slo-2(lf) ( Fig. 5a ). We determined SLO-2 single-channel conductance from the slope of a linear fit to SLO-2 single-channel current amplitudes at the various voltages, and found it to be 117±2 pS in VA5, 120±2 pS in VB6 and 111±2 pS in VD5 ( Fig. 5b ). These values are similar to those of SLO-2 expressed in Xenopus oocytes [23] and in cultured body-wall muscle cells [34] . Next, we analysed the effect of intracellular Cl − on SLO-2 by reducing [Cl − ] from 128.5 to 15.3 mM in the standard pipette solution. This treatment essentially abolished SLO-2 current in WT worms, as suggested by the similar outward current between WT with low [Cl − ] i and slo-2(lf) with high [Cl − ] i , and the lack of an effect of the low [Cl − ] i on outward current in slo-2(lf) ( Fig. 6a ). Finally, we analysed SLO-2 Ca 2+ dependence. In recording the whole-cell current, the concentration of free Ca 2+ in the pipette solution was ~50 nM, which was not expected to cause significant SLO-2 activation [23] . We hypothesized that extracellular Ca 2+ plays a role in SLO-2 activation by establishing Ca 2+ microdomains at the inner openings of Ca 2+ permeable channels, as is the case for mammalian Slo2 activation by extracellular Na + (refs 4 , 5 ). We therefore examined the effects of varying [Ca 2+ ] o between 5 and 0 mM on SLO-2 single-channel activity in outside-out patches with little free Ca 2+ (~50 nM) in the pipette solution. Indeed, SLO-2 activity was high when [Ca 2+ ] o was 5 mM but greatly decreased after [Ca 2+ ] o was changed to 0 mM ( Fig. 6b ). Taken together, our observations suggest that SLO-2 in motor neurons depends on both Cl − and Ca 2+ for activation, and that extracellular Ca 2+ plays an important role in SLO-2 activation. 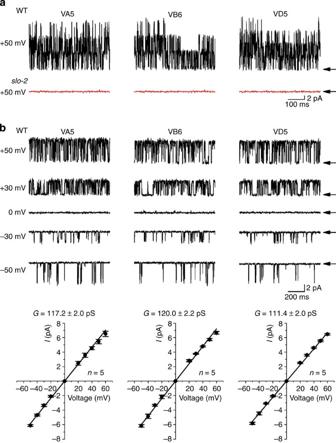Figure 5: Single-channel conductance of motor neuron SLO-2. (a) Sample current traces showing SLO-2 single-channel activities in inside-out patches of wild type and the absence of such activities inslo-2(nf101). (b) Sample SLO-2 single-channel current traces at various membrane voltages from inside-out patches, and the relationship between single-channel current amplitude and holding potential. Data are shown as mean±s.e. SLO-2 single-channel conductance (G) and sample size (n) are shown in the graphs. For display purpose, the sample traces were chosen from regions where only one channel was open. Arrows mark the baseline. The experiments were performed in symmetrical K+(pipette solution III and bath solution as specified in Methods). Figure 5: Single-channel conductance of motor neuron SLO-2. ( a ) Sample current traces showing SLO-2 single-channel activities in inside-out patches of wild type and the absence of such activities in slo-2(nf101) . ( b ) Sample SLO-2 single-channel current traces at various membrane voltages from inside-out patches, and the relationship between single-channel current amplitude and holding potential. Data are shown as mean±s.e. SLO-2 single-channel conductance ( G ) and sample size ( n ) are shown in the graphs. For display purpose, the sample traces were chosen from regions where only one channel was open. Arrows mark the baseline. The experiments were performed in symmetrical K + (pipette solution III and bath solution as specified in Methods). 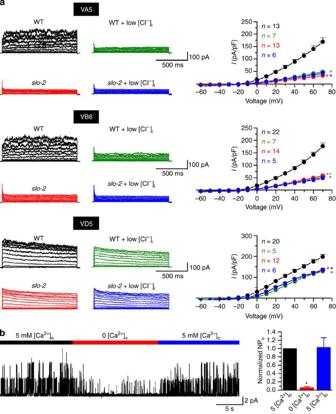Figure 6: SLO-2 activity in motor neurons depends on cytosolic [Cl−] and entry of extracellular Ca2+. (a) Whole-cell current traces and relationships between delayed outward current and voltage in representative motor neurons (VA5, VB6 and VD5) of wild type (WT),slo-2(nf101), WT with low [Cl−] in pipette solution (WT+low [Cl−]i) andslo-2(nf101)with low [Cl−] in pipette solution (slo-2+low [Cl−]i), showing that reducing [Cl−]ifrom the control level (128.5 mM) to a low level (15.3 mM) caused a great reduction of delayed outward current in WT but no change inslo-2(nf101). The asterisk (*) on the right side of a current–voltage relationship indicates a statistically significant (P<0.01) difference compared with WT (two-way mixed model analyses of variance (ANOVA) with Tukey’spost hoctest). All the recordings were performed with extracellular solution I and pipette solution I except for the low [Cl−] experiments, in which pipette solution II was used instead. (b) Effects of varying [Ca2+]oon SLO-2 single-channel activity in outside-out patches at a holding voltage of +30 mV. The open probability (NPo) of SLO-2 was normalized to that of the first 5 mM [Ca2+]operiod. The asterisk (*) indicates a statistically significant difference compared with the first 5 mM [Ca2+]operiod (P<0.01, one-way ANOVA with Tukey’spost hoctest,n=5). The recordings were performed with pipette solution I and either extracellular solution I (5 mM Ca2+) or extracellular solution III (0 Ca2+). In botha,b, data are shown as mean±s.e. Full size image Figure 6: SLO-2 activity in motor neurons depends on cytosolic [Cl − ] and entry of extracellular Ca 2+ . ( a ) Whole-cell current traces and relationships between delayed outward current and voltage in representative motor neurons (VA5, VB6 and VD5) of wild type (WT), slo-2(nf101) , WT with low [Cl − ] in pipette solution (WT+low [Cl − ] i ) and slo-2(nf101) with low [Cl − ] in pipette solution ( slo-2 +low [Cl − ] i ), showing that reducing [Cl − ] i from the control level (128.5 mM) to a low level (15.3 mM) caused a great reduction of delayed outward current in WT but no change in slo-2(nf101) . The asterisk (*) on the right side of a current–voltage relationship indicates a statistically significant ( P <0.01) difference compared with WT (two-way mixed model analyses of variance (ANOVA) with Tukey’s post hoc test). All the recordings were performed with extracellular solution I and pipette solution I except for the low [Cl − ] experiments, in which pipette solution II was used instead. ( b ) Effects of varying [Ca 2+ ] o on SLO-2 single-channel activity in outside-out patches at a holding voltage of +30 mV. The open probability (NP o ) of SLO-2 was normalized to that of the first 5 mM [Ca 2+ ] o period. The asterisk (*) indicates a statistically significant difference compared with the first 5 mM [Ca 2+ ] o period ( P <0.01, one-way ANOVA with Tukey’s post hoc test, n =5). The recordings were performed with pipette solution I and either extracellular solution I (5 mM Ca 2+ ) or extracellular solution III (0 Ca 2+ ). In both a , b , data are shown as mean±s.e. Full size image Ca 2+ entry through EGL-19 is important to SLO-2 activation Given that SLO-2 was activated by Ca 2+ entering the cell, there must be a Ca 2+ channel(s) mediating the Ca 2+ entry. We first examined potential contributions by VGCCs. The C. elegans genome contains three genes encoding the pore-forming α 1 -subunit of VGCCs, including egl-19 (Ca V 1/L-type), unc-2 (Ca V 2/N, P, Q-type) and cca-1 (Ca V 3/T-type) [39] . We selected mutants of these genes for analyses. For unc-2 and cca-1 , we analysed the severe lf or null mutants unc-2(e55) and cca-1(ad1650) (refs 40 , 41 ). For egl-19 , we analysed the gain-of-function mutant egl-19(ad695) and the hypomorphic mutant egl-19(n582) because null mutants die at embryonic stages [42] . Compared with WT, egl-19(ad695) caused a significantly larger delayed outward current in all the motor neurons (VA5, VB6 and VD5), whereas egl-19(n582) showed an opposite effect in VA5 and VB6 ( Fig. 7 ). These effects of the egl-19 mutants were not observed in the presence of slo-2(nf101) ( Fig. 7 ), suggesting that EGL-19 regulates delayed outward current through SLO-2. The insignificant effect of egl-19(n582) on delayed outward current in VD5 ( Fig. 7 ) could be owing to the relatively small SLO-2 current in VD5 ( Fig. 1 ). 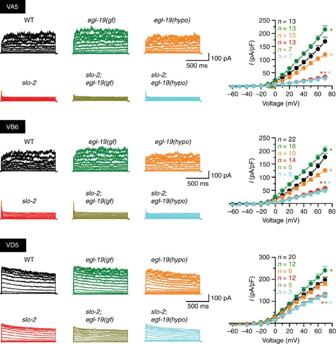Figure 7: Mutations ofegl-19altered delayed outward current of motor neurons in a SLO-2-dependent manner. Whole-cell delayed outward current were recorded from VA5, VB6 and VD5 of wild type (WT),egl-19(ad695)(gain-of-function),egl-19(n582)(hypomorph),slo-2(nf101),slo-2(nf101);egl-19(ad695);andslo-2(nf101);egl-19(n582). Compared with WT,egl-19(ad695)andegl-19(n582)augmented and inhibited delayed outward current, respectively, which were not observed in the presence ofslo-2(nf101). Left: sample current traces in response to voltage steps (−60 to +70 mV at 10 mV intervals) from a holding potential of −60 mV. Right: current–voltage relationships. Data are shown as mean±s.e. The asterisk (*) indicates a statistically significant difference compared with WT (P<0.05, two-way mixed model analyses of variance and Tukey’spost hoctests). The recordings were performed with extracellular solution I and pipette solution I. Figure 7: Mutations of egl-19 altered delayed outward current of motor neurons in a SLO-2-dependent manner. Whole-cell delayed outward current were recorded from VA5, VB6 and VD5 of wild type (WT), egl-19(ad695) (gain-of-function), egl-19(n582) (hypomorph), slo-2(nf101) , slo-2(nf101);egl-19(ad695); and slo-2(nf101);egl-19(n582) . Compared with WT, egl-19(ad695) and egl-19(n582) augmented and inhibited delayed outward current, respectively, which were not observed in the presence of slo-2(nf101) . Left: sample current traces in response to voltage steps (−60 to +70 mV at 10 mV intervals) from a holding potential of −60 mV. Right: current–voltage relationships. Data are shown as mean±s.e. The asterisk (*) indicates a statistically significant difference compared with WT ( P <0.05, two-way mixed model analyses of variance and Tukey’s post hoc tests). The recordings were performed with extracellular solution I and pipette solution I. Full size image Delayed outward current was similar between WT and either unc-2(e55) or cca-1(ad1650) ( Fig. 8 ), suggesting that UNC-2 and CCA-1 do not play a role in SLO-2 activation. In addition to the VGCCs, we assessed potential contributions by several other proteins implicated in either Ca 2+ entry or Ca 2+ release from endoplasmic reticulum, including TRP-1 (canonical transient receptor potential channel) [43] , CLHM-1 (calcium homeostasis modulator, Calhm) [44] , NCA-1 and NCA-2 (putative cation channels) [45] , [46] , and UNC-68 (ryanodine receptor) [47] , [48] by analysing whole-cell current in corresponding mutants. The mutant strains used included trp-1(ok323) (refs 49 , 50 ) , clhm-1(ok3617) (ref. 44 ) , unc-68(r1162) (ref. 47 ) and the double-mutant nca-1(gk9);nca-2(gk5) (refs 45 , 46 , 51 ), which are either nulls or severe lf mutants. Delayed outward current was normal in all these mutants ( Fig. 8 ). Taken together, the aforementioned observations suggest that EGL-19 is likely the primary, if not the only, Ca 2+ channel mediating SLO-2 activation in motor neurons. 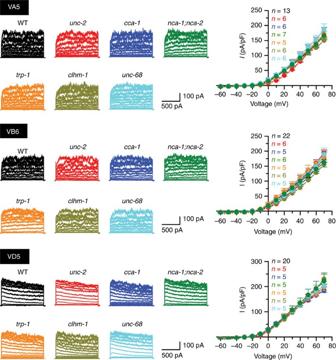Figure 8: Delayed outward current was normal in mutants of other Ca2+channels. Delayed outward currents were unchanged inunc-2(e55),cca-1(ad1650),trp-1(ok323),clhm-1(ok3617),unc-68(r1162)and the double-mutantnca-1(gk9);nca-2(gk5)compared with wild type (WT; two-way mixed model analyses of variance). Left: sample current traces in response to voltage steps (−60 to +70 mV at 10 mV intervals) from a holding potential of −60 mV. Right: current–voltage relationships. Data are shown as mean±s.e. The recordings were performed with extracellular solution I and pipette solution I. Figure 8: Delayed outward current was normal in mutants of other Ca 2+ channels. Delayed outward currents were unchanged in unc-2(e55) , cca-1(ad1650) , trp-1(ok323) , clhm-1(ok3617) , unc-68(r1162) and the double-mutant nca-1(gk9);nca-2(gk5) compared with wild type (WT; two-way mixed model analyses of variance). Left: sample current traces in response to voltage steps (−60 to +70 mV at 10 mV intervals) from a holding potential of −60 mV. Right: current–voltage relationships. Data are shown as mean±s.e. The recordings were performed with extracellular solution I and pipette solution I. Full size image Our electrophysiological data indicate that SLO-2 is the primary contributor to delayed outward current in A and B class motor neurons, and one of two major contributors to this current in D class motor neurons. These observations are reminiscent of those with rat central neurons where Slo2 channels contribute to a large portion of delayed outward current [4] , [5] , [6] . The similar observations with rat and C. elegans suggest that these channels began to assume the important task of conducting delayed outward current early in evolution, and that their existence has been indispensable. The resting membrane potential of mammalian neurons is generally close to the K + equilibrium potential owing to the function of background K + channels. Two-pore domain K + (K2P) channels appear to be important molecular entities of the background K + channels because they are largely voltage independent [52] . The C. elegans genome has 46 K2P genes [33] . Although no experimental evidence is currently available, it is conceivable that some of these channels may play roles in setting the resting membrane potential. The present study shows that SLO-2, which is not a K2P channel, plays an important role in setting the resting membrane potential of motor neurons. A similar role of SLO-2 has been observed in C. elegans body-wall muscle [25] . Thus, SLO-2 might be important in setting the resting membrane potential of many C. elegans neurons and muscle cells. slo-2 mutation resulted in a longer duration and a larger persistent current of PSC bursts compared with WT, suggesting that a physiological function of SLO-2 is to shorten the duration and decrease the charge transfer rate of PSC bursts. SLO-2 likely performs these physiological functions by regulating neurotransmitter release because body-wall muscle sensitivities to neurotransmitters are normal in slo-2 mutant. Given that PSC bursts are the physiological signals used by motor neurons to control body-wall muscle cells [27] , SLO-2 likely plays an important role in regulating muscle function. This physiological function of SLO-2 could be related to its effect on the resting membrane potential of motor neurons and its interactions with other proteins such as EGL-19. The substantial decrease of SLO-2 single-channel activity in outside-out patches following the removal of Ca 2+ on the extracellular side suggests that SLO-2 activity depends on Ca 2+ entry. EGL-19 appeared to play an important role in SLO-2 activation as SLO-2 current was significantly increased in egl-19(gf) but decreased in egl-19(hypomorph) . Indeed, EGL-19 might be the only channel with this function given that mutants of a variety of other genes known to be important to either entry of extracellular Ca 2+ or release of Ca 2+ from the endoplasmic reticulum did not show a change of SLO-2 current. The coupling of SLO-2 activation to Ca 2+ entry through EGL-19 explains why large SLO-2 current is observed in C. elegans motor neurons in whole-cell voltage-clamp experiments with little free Ca 2+ in the pipette solution. The dependence of SLO-2 activity on EGL-19 is analogous to that of mammalian Slo2 on tetrodotoxin-sensitive Na + channels [4] , [5] . C. elegans does not have any genes encoding voltage-gated Na + channels and likely uses Ca 2+ exclusively for carrying excitatory inward current [39] , which is in contrast to mammals in which Na + action potentials generally underlie cellular excitability. It thus appears that coupling channel activation to the entry of a cation is a conserved property of SLO-2/Slo2 channels, but evolution has tuned this property to match the dominant ion used in cellular excitation in each species. The C. elegans Slo family of K + channels includes two members: SLO-1 and SLO-2 (refs 24 , 33 ). slo-1(lf) also prolongs the duration of PSC bursts [27] . However, there are major differences in synaptic phenotypes between slo-1 and slo-2 mutants. Unlike slo-2(lf) , slo-1(lf) does not alter the persistent current of PSC bursts but may cause larger evoked PSC amplitude at the C. elegans NMJ compared with WT [27] , [37] , [53] . Thus, SLO-1 and SLO-2 likely inhibit neurotransmitter release through somewhat different mechanisms, which could be related to their different subcellular localization and/or functional coupling to different VGCCs. While SLO-1 is localized at the presynaptic site [53] and is likely regulated by Ca 2+ entry through UNC-2, which is also localized at the presynaptic site [54] , SLO-2 might be localized to other subcellular domains and coupled to Ca 2+ entry through EGL-19. SLO-1 did not show a detectable contribution to the whole-cell current of motor neurons in spite of its important role in regulating neurotransmitter release. There are two possible causes for this discrepancy. First, the free [Ca 2+ ] of the recording pipette (~50 nM) was insufficient to allow significant SLO-1 activation. Second, SLO-1 current at presynaptic sites, which could potentially result from a coupling to Ca 2+ entry through UNC-2, might have been shunted before reaching the soma. We have noted a similar discrepancy between SLO-1 function and its contribution to whole-cell current in C. elegans body-wall muscle, where SLO-1 is expressed [36] and plays an important role in regulating Ca 2+ transients [53] , but whole-cell current was indistinguishable between WT and slo-1 null mutant even when a pipette solution containing 20 μM free Ca 2+ concentration was used in the recording (unpublished observation). slo-2 mutant worms displayed no obvious locomotion defects, which is somewhat surprising given that SLO-2 is an important K + channel in both body-wall muscle cells [15] , [25] , [34] and motor neurons. This is analogous to the movement phenotypes of slo-1 mutants. Although SLO-1 also plays important physiological roles in both neurons [36] , [55] and body-wall muscle cells [56] , [57] , [58] , slo-1 mutants only show a slightly larger head bending angle compared with WT, which results from SLO-1 deficiency in body-wall muscle cells, and may be detected only by either a trained observer or computer-based analyses [59] , [60] . Perhaps potential effects of SLO-2 deficiency on behavioural phenotypes would become more obvious in a sensitized genetic background or under some specific conditions such as hypoxia [15] . The original paper on SLO-2 reported that SLO-2 heterologously expressed in Xenopus oocytes is activated by Cl − on the intracellular side [23] . Consistently, the concentration of Cl − in the recording pipette solution was found to have a large effect on SLO-2 activity of C. elegans body-wall muscle cells in situ [34] . However, the Cl − dependence of SLO-2 was challenged by a recent study showing that at least two isoforms of SLO-2, including the original one used in the heterologous expression experiments, are Cl − insensitive [38] . It was suggested that the apparent Cl − dependence of SLO-2 observed in the earlier study reflected contamination by an endogenous Cl − current present in Xenopus oocytes [38] . Our observations provide evidence that SLO-2 in native motor neurons is a Cl − -sensitive channel. Both the human genome and C. elegans genome contain over 70 potassium channel genes [33] , [61] . The fact that SLO-2/Slo2 channels play a major role in conducting delayed outward current in neurons of both species suggests that this subfamily of K + channels likely performs conserved physiological functions of unusual importance. It will be interesting to know whether mammalian Slo2 channels also control the resting membrane potential and regulate synaptic transmission, and how their physiological functions are modulated in vivo . Since knockout mice of both Slo2 genes ( KCNT1 and KCNT2 ) are now available from the Jackson laboratory (MGI:1924627 and 3036273), it is desirable to compare between WT and the knockout mice the resting membrane potential and PSCs in selected central neurons. In addition, many Slo2 mutations identified in human epileptic patients may be introduced into worm SLO-2 to investigate how these mutations affect channel function and/or expression in vivo . In some cases, expression of a mutated channel may cause an obvious behavioural phenotype, which could serve as a very useful tool for identifying conserved Slo2 channel regulatory proteins through mutant screen in this genetically tractable model organism. C. elegans culture and strains C. elegans hermaphrodites were raised on nematode growth medium plates spotted with a layer of OP50 Escherichia coli at 21 °C inside an environmental chamber. The strains used included WT (Bristol N2), slo-2(nf101) , shk-1(ok1581) , shl-1(ok1168) , slo-1(md1745) , egl-19(ad695) , egl-19(n582) , unc-2(e55) , cca-1(ad1650) , nca-1(gk9);nca-2(gk5) , trp-1(ok323) , clhm-1(ok3617) , unc-68(r1162) , slo-2(nf101);shk-1(ok1581) , slo-2(nf101);egl-19(ad695) and slo-2(nf101);egl-19(n582) . Mutant rescue Neuron-specific rescue was performed by injecting a plasmid containing the pan-neuronal P rab-3 and full-length slo-2b cDNA (F08B12.3b; www.wormbase.org ) [23] fused in-frame at its 3′-end to GFP coding sequence into slo-2(nf101) using a standard technique [62] . Electrophysiology All electrophysiological experiments were performed with adult hermaphrodites. An animal was immobilized on a glass coverslip by applying Vetbond M Tissue Adhesive (3M Company, St Paul, MN, USA). Application of the glue was generally restricted to the dorsal anterior portion (excluding the head) of the animal, allowing the head and tail to sway freely during the experiment. A short (~300 μm) longitudinal incision was made along the glued region. After clearing the viscera by suction through a glass pipette, the cuticle flap was folded back and glued to the coverslip, thereby exposing several ventral body-wall muscle cells and a small number of motor neurons anterior to the vulva. Borosilicate glass pipettes were used as electrodes for recording whole-cell and single-channel currents. Pipette tip resistance for recording muscle cell current was 3–5 MΩ, whereas that for recording motor neuron current was ~20 MΩ. The dissected worm preparation was treated briefly with collagenase A (0.5 mg ml −1 for 10–15 s; Roche Applied Science, catalogue number 10103578001) and perfused with the extracellular solution for 5- to 10-fold of bath volume. Classical whole-cell configuration was obtained by applying a negative pressure to the recording pipette. Inside-out patches were obtained by quickly pulling away the recording pipette after the formation of a gigaohm seal, whereas outside-out patches were obtained by slowly pulling away the recording pipette after achieving the whole-cell configuration. Current- and voltage-clamp experiments were performed with a Multiclamp 700B amplifier (Molecular Devices, Sunnyvale, CA, USA) and the Clampex software (version 10, Molecular Devices). Data were sampled at a rate of 10 kHz after filtering at 2 kHz. Spontaneous membrane potential changes were recorded using the current-clamp technique without current injection. Motor neuron whole-cell outward currents were recorded by applying a series of voltage steps (−60 to +70 mV at 10-mV intervals, 1,200 ms pulse duration) from a holding potential of −60 mV. Evoked PSC, spontaneous PSC and exogenous ACh- or GABA-induced PSC were recorded from body-wall muscle cells at a holding potential of −60 mV. Evoked PSC was caused by applying an electric stimulus at a saturating strength (20 V, 0.5 ms) through a glass pipette electrode placed near the ventral nerve cord. The stimulus was generated by a square pulse stimulator (S48, Grass Technologies, Warwick, RI, USA). To obtain representative evoked PSC from each preparation, the position of the electrode was adjusted until a maximal evoked PSC peak amplitude was observed. Muscle responses to exogenous ACh and GABA were caused by puffing the chemicals (100 μM) through a glass pipette using a FemtoJet injector (Eppendorf) with the pressure pulse set at 0.2 p.s.i. and 0.1 s. Solutions Three different extracellular solutions and three different pipette solutions were used, as specified in figure legends. Extracellular solution I contained (in mM) 140 NaCl, 5 KCl, 5 CaCl 2 , 5 MgCl 2 , 11 dextrose and 5 HEPES (pH 7.2). Extracellular solution II differed from extracellular solution I in that CaCl 2 was reduced to 0.5 mM. Extracellular solution III differed from extracellular solution I in that CaCl 2 was eliminated, 5 mM EGTA was added and NaCl was increased to 150 mM. Pipette solution I contained (in mM) 120 KCl, 20 KOH, 5 Tris, 0.25 CaCl 2 , 4 MgCl 2 , 36 sucrose, 5 EGTA and 4 Na 2 ATP (pH 7.2). Pipette solution II differed from pipette solution I in that 113.2 KCl was substituted by K + gluconate. Pipette solution III contained (in mM) 150 K + gluconate, 1 Mg 2+ gluconate and 10 HEPES (pH 7.2). The bath solution used in inside-out patch experiments contained (in mM) 100 K + gluconate, 50 KCl, 1 Mg 2+ gluconate, 0.1 Ca 2+ gluconate and 10 HEPES (pH 7.2). Data analyses Amplitudes of whole-cell current in response to voltage steps were determined from the mean current during the last 100 ms of the 1,200-ms voltage pulses using the Clampfit software (version 10, Molecular Devices). SPSS software (IBM Corp., New York, USA) was used for comparing the current among different genotypes by two-way mixed model analyses of variance. In these analyses, voltage steps were treated as within-subject variables, whereas genotypes as between-subject variables. Tukey’s post hoc tests were used to determine whether a statistically significant difference exists between specified genotypes. All genotypes shown in Figs 1 and 6 , 7 , 8 were analysed together so that valid statistical comparisons could be made among them. SLO-2 single-channel amplitude and open probability were quantified using Clampfit. PSC bursts were identified as an apparent increase in PSC frequency with a persistent current lasting >3 s (ref. 27 ). The duration, mean persistent current amplitude and mean charge transfer rate of PSC bursts were determined with Clampfit. The frequency and amplitude of spontaneous PSCs were quantified using MiniAnalysis (Synaptosoft, Inc., Decatur, GA, USA) with the detection threshold set at 10 pA for initial automatic event detection, followed by visual inspections to include missed events (≥5 pA) and to exclude false events resulting from baseline fluctuations. The software was set to search for a baseline 3 ms before a PSC event and use the average of a 1-ms period as the baseline level. Peak amplitudes of evoked PSCs and of muscle responses to exogenous ACh or GABA were quantified using Clampfit. The average of the largest two evoked PSCs recorded from each muscle cell was used for statistical comparisons. Upstate was defined as a sudden increase (>5 mV) in the membrane potential lasting longer than 3 s. Upstate potential was the mean membrane voltage during the upstate (quantified with Clampfit), whereas upstate amplitude was the voltage difference between upstate potential and the resting membrane potential. All the upstates of each recording (3–5 min) were analysed to obtain an averaged value of each parameter (for example, amplitude and duration) before statistical analyses. Statistical comparisons were performed with OriginPro (version 9, OriginLab, Northampton, MA, USA) using either one-way analyses of variance or unpaired t -test (depending on whether there were >2 groups). All values are shown as mean±s.e. P <0.05 is considered to be statistically significant. The sample size ( n ) equals the number of cells or membrane patches analysed. Data graphing was performed with OriginPro. How to cite this article: Liu, P. et al . SLO-2 potassium channel is an important regulator of neurotransmitter release in Caenorhabditis elegans . Nat. Commun. 5:5155 doi: 10.1038/ncomms6155 (2014).